Nanomechanical DNA origami 'single-molecule beacons' directly imaged by atomic force microscopy DNA origami involves the folding of long single-stranded DNA into designed structures with the aid of short staple strands; such structures may enable the development of useful nanomechanical DNA devices. Here we develop versatile sensing systems for a variety of chemical and biological targets at molecular resolution. We have designed functional nanomechanical DNA origami devices that can be used as 'single-molecule beacons', and function as pinching devices. Using 'DNA origami pliers' and 'DNA origami forceps', which consist of two levers ~170 nm long connected at a fulcrum, various single-molecule inorganic and organic targets ranging from metal ions to proteins can be visually detected using atomic force microscopy by a shape transition of the origami devices. Any detection mechanism suitable for the target of interest, pinching, zipping or unzipping, can be chosen and used orthogonally with differently shaped origami devices in the same mixture using a single platform. The rapid development of nanotechnology has enabled the precise manipulation of nanomaterials. However, typical analytical methods for chemical or biochemical targets are still based on spectroscopic principles, which reflect the average behaviour of a vast number of molecules. To analyse the behaviour of an individual molecule, nanomechanical devices that can work with target molecules in a single-molecule manner are required. Structural DNA nanotechnology [1] , [2] , [3] , based on the programmed assembly of branched DNA helices, is a key technology that can provide such functional nanomechanical devices. DNA devices such as DNA tweezers [4] , [5] , [6] , DNA scissors [7] , [8] , and DNA walkers have been constructed [9] , [10] , [11] , [12] , [13] and used as molecular sensors for various targets [14] , [15] , following the success of molecular beacons [16] , [17] . However, individual molecules of these devices are still too small to be easily analysed at molecular resolution using current microscopy techniques. DNA origami [18] , [19] , [20] , [21] , in which long single-stranded DNA is folded into a designed nanostructure with the aid of many short staple strands, is a powerful new tool in structural DNA nanotechnology that provides robust and precise nanostructures in both 2D and 3D that are visible through atomic force microscopy (AFM) or electron microscopy. Taking advantage of their precise addressability at nanometre resolution, some custom nano-instruments for studying single-molecule interactions in biology and chemistry, using DNA origami assembly as a nanoscale stage, have recently been proposed [22] , [23] , [24] . Despite these properties, only a limited number of studies have been published on DNA origami as a building material for nanomechanical DNA devices [25] , [26] ; some recent reports have discussed its usefulness as a scaffold on which nanomechanical DNA devices could be located [27] , [28] , [29] . Here we present functional nanomechanical DNA origami devices that can be used as versatile and visible 'single-molecule beacons' ( Fig. 1 ). Using 'DNA origami pliers' and 'DNA origami forceps' ( Fig. 2 ) that consist of two levers of ~170 nm in length connected at a fulcrum, various inorganic/organic targets, from metal ions to proteins, were visually detected in a single-molecule manner as a shape transition of DNA origami devices, using AFM. 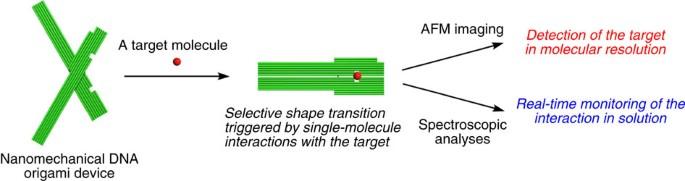Figure 1: Detection of various targets using DNA origami devices. The selective shape transitions of DNA origami devices triggered by intermolecular interactions with the target are visualized at molecular resolution using AFM on mica or monitored in real-time by fluorescence measurement in solution. Figure 1: Detection of various targets using DNA origami devices. The selective shape transitions of DNA origami devices triggered by intermolecular interactions with the target are visualized at molecular resolution using AFM on mica or monitored in real-time by fluorescence measurement in solution. 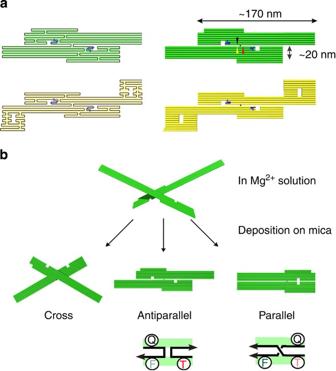Figure 2: Structure of nanomechanical DNA origami devices. (a) Folding patterns of M13 scaffold in DNA origami pliers and DNA origami forceps with extra finger-hole-like structure (lower left) for visual discrimination of coexisting targets in solution. Staple strands are omitted, except for the anchor strands with extra 8-nucleotide toeholds (presented in blue). Illustrations at right represent the approximate size of DNA helices, levers and concavities. The two levers are joined at a fulcrum through two phosphodiester bonds in the M13 scaffold so that an immobile Holliday junction is formed. Yellow, red, and black wedges indicate the positions of fluorescent dyes and a quencher (see below). (b) Expected solution structure of DNA pliers and three possible forms: cross, antiparallel, and parallel closed, observed on mica. The configuration of the M13 scaffold (drawn in black lines) at the fulcrum is shown below. To monitor the structure of origami devices in solution, one of the levers of the DNA pliers was fluorescently labelled with 6-fluoresceincarboxyamide (yellow wedge; F, FAM) and Texas Red (red wedge; T, TXR) at two sites one and a half helical turns away from the fulcrum. The other lever was modified with a Black hole quencher-2 (black wedge, Q, BHQ-2) group so that the fluorescence of FAM would be quenched by nearby BHQ-2 when DNA pliers were in antiparallel form. The shape transition of the pliers into parallel form brings BHQ-2 closer to TXR than FAM, resulting in the quenching of TXR and recovery of FAM emission. Full size image Figure 2: Structure of nanomechanical DNA origami devices. ( a ) Folding patterns of M13 scaffold in DNA origami pliers and DNA origami forceps with extra finger-hole-like structure (lower left) for visual discrimination of coexisting targets in solution. Staple strands are omitted, except for the anchor strands with extra 8-nucleotide toeholds (presented in blue). Illustrations at right represent the approximate size of DNA helices, levers and concavities. The two levers are joined at a fulcrum through two phosphodiester bonds in the M13 scaffold so that an immobile Holliday junction is formed. Yellow, red, and black wedges indicate the positions of fluorescent dyes and a quencher (see below). ( b ) Expected solution structure of DNA pliers and three possible forms: cross, antiparallel, and parallel closed, observed on mica. The configuration of the M13 scaffold (drawn in black lines) at the fulcrum is shown below. To monitor the structure of origami devices in solution, one of the levers of the DNA pliers was fluorescently labelled with 6-fluoresceincarboxyamide (yellow wedge; F, FAM) and Texas Red (red wedge; T, TXR) at two sites one and a half helical turns away from the fulcrum. The other lever was modified with a Black hole quencher-2 (black wedge, Q, BHQ-2) group so that the fluorescence of FAM would be quenched by nearby BHQ-2 when DNA pliers were in antiparallel form. The shape transition of the pliers into parallel form brings BHQ-2 closer to TXR than FAM, resulting in the quenching of TXR and recovery of FAM emission. Full size image The design of nanomechanical DNA origami devices The DNA origami devices used in this study behave like nano-sized pinching devices ( Fig. 1 ). Shape transitions of nanomechanical DNA origami devices, such as the closing or opening of pliers, are selectively triggered by interactions with target molecules and visualized using AFM imaging. The existence of the target is therefore determined at molecular resolution. This sensing method is applicable to versatile targets because a variety of interactions (for example, protein–ligand, DNA–RNA, or DNA–metal ions) can be employed. Figure 2 shows the detailed structure of the DNA origami devices used in this study. The first origami device shown is the 'DNA origami pliers' ( Fig. 2a ), which consist of two ca. 170-nm lever domains, each of which is made of six antiparallel DNA helices from a part of M13 scaffold and 117 staple strands (ca. 20 nm wide). These levers are joined together at a fulcrum via two phosphodiester linkages in the M13 scaffold to form an immobile Holliday junction. In a Mg 2+ solution, typically used in DNA origami preparation, the DNA four-way junction is known to be a right-handed, antiparallel stacked X-structure with a small angle of 60° (refs 31 , 31 , 32 ). DNA origami pliers in solution are thus expected to be twisted, as illustrated in Figure 2b . AFM measurements of DNA origami devices require deposition on a mica surface. Origami devices adhered to the 2D surface can adopt three forms. The most likely form is a 'cross', which most closely resembles the expected twisted structure of the origami pliers. The second feasible structure is an 'antiparallel form', in which two levers are aligned in parallel on a plane but point in opposite directions. Configuration of the M13 scaffold at the fulcrum in this form is in 'antiparallel' mode, which is rather relaxed, and is a typical configuration in DNA origami design. The third feasible form is a 'parallel closed form' in which the levers are parallel. This configuration of the DNA four-way junction at the fulcrum is considered unfavourable compared with the antiparallel mode [30] , [31] , [32] . Thus, origami devices in the parallel closed form are expected to be the least populated species in the AFM images unless some further interaction rotates the fulcrum. Each of the levers has a small concavity two helical turns long and two helices wide (ca. 7 nm×7 nm). These concavities serve as the jaws of pliers that pinch the target molecule. When DNA pliers are in the parallel closed form, these concavities lie next to each other to form a larger cavity that accommodates the pinched target stably during AFM scanning, as shown in our previous studies [33] , [34] . The shape transition of DNA pliers in the presence of their targets is triggered by three independent mechanisms: 'pinching' ( Fig. 3 ), 'zipping' ( Fig. 4 ), and 'unzipping' ( Fig. 5 ). 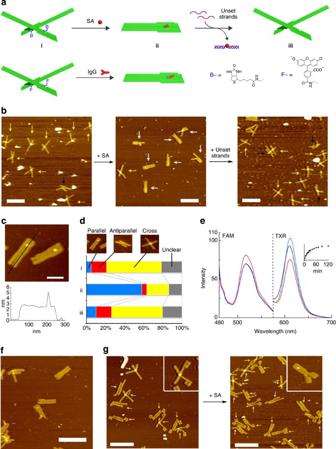Figure 3: Single-molecule pinching of proteins. (a) Schematic illustration of SA and IgG pinching. (b) AFM images for SA pinching and release by biotinylated DNA pliers. The scale bars are 300 nm. The dominant form of DNA pliers in Mg2+solution before SA addition (left ina, i) was a cross (yellow arrows). After SA addition (middle ina, ii), DNA pliers selectively pinched exactly one SA tetramer and closed into the parallel closed form (white arrows). The population of DNA pliers in the cross form recovered significantly when the biotinylated anchor strands, together with SA, were selectively detached from the DNA pliers (right ina, iii). DNA pliers in the antiparallel form (black arrows) were always a minor species. (c) A height profile of parallel DNA pliers with SA (black line in the image). The scale bar is 100 nm. (d) Form distribution at each step ina, estimated by counting the motifs in AFM images. (e) Fluorescence spectra of doubly dye-labelled DNA pliers before (left ina, green) and 10 min after SA addition (middle ina, red) and 2 h after the addition of unset strands at room temperature (right ina, blue). The excitation wavelengths for 6-fluoresceincarboxyamide (FAM, 460–575 nm) and Texas Red, (TXR, 575–700 nm) spectra were 450 and 550 nm, respectively. Inset, time course of the recovery of TXR emission at 612 nm after the addition of unset strands (from the red spectrum to the blue one). (f) Single-molecule pinching of anti-fluorescein IgG by FAM-modified DNA pliers. The scale bar is 300 nm. Slightly lower objects than SA (3–4 nm) were observed in the jaws. (g) Selective pinching of SA by biotinylated DNA forceps (white arrows) in a mixture with FAM-labelled DNA pliers (yellow arrows). The scale bars are 300 nm. The insets show zoomed images of typical DNA forceps. Figure 3: Single-molecule pinching of proteins. ( a ) Schematic illustration of SA and IgG pinching. ( b ) AFM images for SA pinching and release by biotinylated DNA pliers. The scale bars are 300 nm. The dominant form of DNA pliers in Mg 2+ solution before SA addition (left in a , i) was a cross (yellow arrows). After SA addition (middle in a , ii), DNA pliers selectively pinched exactly one SA tetramer and closed into the parallel closed form (white arrows). The population of DNA pliers in the cross form recovered significantly when the biotinylated anchor strands, together with SA, were selectively detached from the DNA pliers (right in a , iii). DNA pliers in the antiparallel form (black arrows) were always a minor species. ( c ) A height profile of parallel DNA pliers with SA (black line in the image). The scale bar is 100 nm. ( d ) Form distribution at each step in a , estimated by counting the motifs in AFM images. ( e ) Fluorescence spectra of doubly dye-labelled DNA pliers before (left in a , green) and 10 min after SA addition (middle in a , red) and 2 h after the addition of unset strands at room temperature (right in a , blue). The excitation wavelengths for 6-fluoresceincarboxyamide (FAM, 460–575 nm) and Texas Red, (TXR, 575–700 nm) spectra were 450 and 550 nm, respectively. Inset, time course of the recovery of TXR emission at 612 nm after the addition of unset strands (from the red spectrum to the blue one). ( f ) Single-molecule pinching of anti-fluorescein IgG by FAM-modified DNA pliers. The scale bar is 300 nm. Slightly lower objects than SA (3–4 nm) were observed in the jaws. ( g ) Selective pinching of SA by biotinylated DNA forceps (white arrows) in a mixture with FAM-labelled DNA pliers (yellow arrows). The scale bars are 300 nm. The insets show zoomed images of typical DNA forceps. 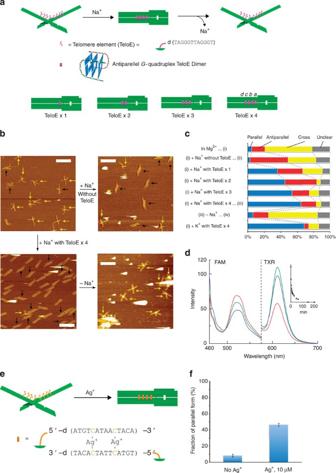Figure 4: Metal ion detection by zipping mechanism. (a) Schematic illustration of Na+-triggered zipping of DNA pliers bearing a G-quadruplex zipper. The four modified sites are indicated below. (b) AFM images for Na+-sensing. Un-indexed DNA pliers in the images are all in the parallel form. For the pliers without any TeloE, a significant increase in antiparallel DNA pliers (black arrows) was observed in a solution containing an extra 200 mM Na+(top right) compared with the solution containing 12.5 mM Mg2+alone (top left). For DNA pliers bearing four TeloE on the levers, on the other hand, most of the pliers were found in the parallel closed form, and few crosses (yellow arrows) were observed (bottom left). Most of the parallel closed pliers in opened up again when Na+was removed from the solution (bottom right). (c) Form distribution of DNA pliers estimated by counting the motifs in AFM images. Concentration of K+in the bottom was 100 mM. (d) Fluorescence spectra before (green) and 2 h after (red) Na+addition at room temperature and after Na+removal (blue). Inset, time course of the quenching of TXR emission at 612 nm after the addition of Na+to the solution (from the green spectrum to the red one). (e) Zipper elements involving C–C mismatches used for Ag+detection. (f) Ag+detection by DNA pliers bearing C–C mismatched zipper elements. Almost 47% of the clearly resolved DNA pliers (n=138) were in the parallel closed form after the addition of Ag+to the solution (final concentration, 10 μM), whereas parallel pliers represented only 8% (n=111) of DNA pliers in the solution without Ag+. The error bars indicate the standard errors. Full size image Figure 4: Metal ion detection by zipping mechanism. ( a ) Schematic illustration of Na + -triggered zipping of DNA pliers bearing a G-quadruplex zipper. The four modified sites are indicated below. ( b ) AFM images for Na + -sensing. Un-indexed DNA pliers in the images are all in the parallel form. For the pliers without any TeloE, a significant increase in antiparallel DNA pliers (black arrows) was observed in a solution containing an extra 200 mM Na + (top right) compared with the solution containing 12.5 mM Mg 2+ alone (top left). For DNA pliers bearing four TeloE on the levers, on the other hand, most of the pliers were found in the parallel closed form, and few crosses (yellow arrows) were observed (bottom left). Most of the parallel closed pliers in opened up again when Na + was removed from the solution (bottom right). ( c ) Form distribution of DNA pliers estimated by counting the motifs in AFM images. Concentration of K + in the bottom was 100 mM. ( d ) Fluorescence spectra before (green) and 2 h after (red) Na + addition at room temperature and after Na + removal (blue). Inset, time course of the quenching of TXR emission at 612 nm after the addition of Na + to the solution (from the green spectrum to the red one). ( e ) Zipper elements involving C–C mismatches used for Ag + detection. ( f ) Ag + detection by DNA pliers bearing C–C mismatched zipper elements. Almost 47% of the clearly resolved DNA pliers ( n =138) were in the parallel closed form after the addition of Ag + to the solution (final concentration, 10 μM), whereas parallel pliers represented only 8% ( n =111) of DNA pliers in the solution without Ag + . The error bars indicate the standard errors. 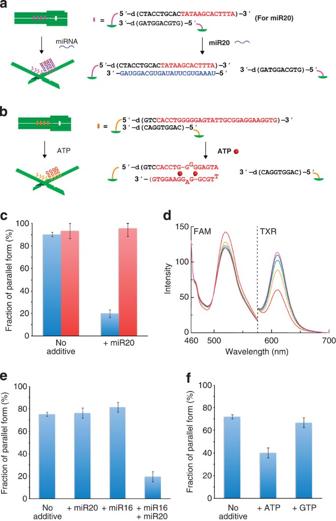Figure 5: Detection of small molecules by unzipping mechanism. Detection of miRNA was performed using a selective strand displacement technique (a). ATP detection was done using aptamer-based elements (b). (c) Selective detection of human miR20 (final concentration, 200 nM) with miR20-targeting DNA pliers (blue bars) in a 1:1 mixture with miR16-targeting DNA forceps (red bars). The error bars indicate the standard errors (n=80 and 55 for DNA pliers before and after miR20 addition, respectively, andn=44 for DNA forceps in both of the systems). (d) Fluorescence spectra of dual-labelled miR20-targeting DNA pliers before (red) and 1 (orange), 2 (green), 3 (blue), and 4 (magenta) hours after miR20 addition at room temperature. (e) AND detection of two miRNA targets using miR20 and miR16 dual-targeting DNA pliers. Addition of only one of the two targets to the solution did not alter the fraction of parallel closed pliers (n=127 for miR20 and 113 for miR16) from the value before addition (n=121). Only when both targets were added was a significant decrease of the fraction observed (n=137). The error bars indicate the standard errors. (f) ATP detection by DNA pliers bearing aptamer-based zipper elements. The initial yield of parallel pliers after annealing was 72% (n=199). After ATP was added to the solution (final concentration, 1 mM), the yield decreased to 40% (n=217), whereas the addition of GTP did not affect the yield significantly (66%,n=126). The error bars indicate the standard errors. Full size image Figure 5: Detection of small molecules by unzipping mechanism. Detection of miRNA was performed using a selective strand displacement technique ( a ). ATP detection was done using aptamer-based elements ( b ). ( c ) Selective detection of human miR20 (final concentration, 200 nM) with miR20-targeting DNA pliers (blue bars) in a 1:1 mixture with miR16-targeting DNA forceps (red bars). The error bars indicate the standard errors ( n =80 and 55 for DNA pliers before and after miR20 addition, respectively, and n =44 for DNA forceps in both of the systems). ( d ) Fluorescence spectra of dual-labelled miR20-targeting DNA pliers before (red) and 1 (orange), 2 (green), 3 (blue), and 4 (magenta) hours after miR20 addition at room temperature. ( e ) AND detection of two miRNA targets using miR20 and miR16 dual-targeting DNA pliers. Addition of only one of the two targets to the solution did not alter the fraction of parallel closed pliers ( n =127 for miR20 and 113 for miR16) from the value before addition ( n =121). Only when both targets were added was a significant decrease of the fraction observed ( n =137). The error bars indicate the standard errors. ( f ) ATP detection by DNA pliers bearing aptamer-based zipper elements. The initial yield of parallel pliers after annealing was 72% ( n =199). After ATP was added to the solution (final concentration, 1 mM), the yield decreased to 40% ( n =217), whereas the addition of GTP did not affect the yield significantly (66%, n =126). The error bars indicate the standard errors. Full size image Detection of proteins by pinching mechanism Pinching is a process that detects single-target molecules that bind to multiple ligands each ( Fig. 3a ). For this purpose, two ligands are attached to each of the staple strands placed in the concavities (anchor strands, drawn in blue in Fig. 2a ), and these ligands cooperatively capture a single-target molecule between the jaws. This intramolecular process triggers a shape transition in the origami device from the cross or antiparallel form to the parallel closed form, which can be visualized using AFM imaging or monitored in solution using spectroscopic analyses. Figure 3b shows typical AFM images of selective, single-molecule pinching of a streptavidin tetramer (SA), which strongly binds to four biotin groups, using DNA origami pliers. Here the DNA pliers were modified with a biotin group in each of the jaws. The dominant species initially observed in 1×TAE/Mg 2+ buffer solution without SA (left, i) was DNA pliers in cross (58% yield), which is consistent with the X-structure of the DNA four-way junction. The population of DNA pliers in antiparallel form was 16%; only 5% of DNA pliers were in the parallel closed form. The preference for the antiparallel over the parallel closed form was in accordance with previous observations. When SA was added to the solution, the populations were drastically altered. Almost 58% of DNA pliers were found in the parallel closed form in the presence of SA (middle). As shown in Figure 3c , a bright spot 5 nm in height, which corresponds to the expected diameter of the pinched SA molecule, was found in the jaws of most of the parallel pliers. The yields of antiparallel and cross pliers in the presence of SA were 5 and 23%, respectively. Spectroscopic analyses have shown that the parallel pliers observed under AFM were formed in solution before deposition, triggered by SA addition. As shown in Figure 3e , the fluorescence spectra of doubly dye-labelled DNA pliers (see Fig. 2 ) showed a significant quenching of TXR emission (ca. 23% at 612 nm) and an enhancement of FAM emission (ca. 17% at 517 nm) immediately after the addition of one equivalent of SA to the solution. The only reasonable explanation for such a drastic shape change is that the single SA tetramer bridged the two levers by binding the attached biotins. The potential for nanomechanical DNA origami as a single-molecule detector for noncovalent and multidentate biochemical interactions has thus been shown. To further prove that the shape transition to parallel pliers was achieved solely by biotin–SA–biotin bidentate binding, the biotinylated anchor strands were selectively detached from the DNA pliers after SA pinching using a DNA strand displacement technique with the aid of the extra 8-nucleotide toehold sequence on the anchor strands (right in Fig. 3b ) [4] . After 2 h incubation at room temperature in the presence of 10 equivalents of unset strands complementary to the anchor strands, the population of parallel pliers decreased to 10%, and pliers in the cross form became the dominant species (53%) again as expected. Recovery of TXR emission to ca. 90% of the initial intensity and nearly complete re-quenching of FAM emission was also consistent with the AFM measurements ( Fig. 3e ). As we recently showed through SA nanopatterning on a punched DNA origami scaffold [35] , repetitive cycles of pinching and release are possible through the readdition of anchor and then unset strands. The target molecules that can be pinched by DNA origami devices are not limited to SA. When FAM-modified anchor strands were used in place of biotinylated anchor strands, DNA pliers selectively pinched anti-fluorescein IgG in the jaws and adopted the parallel closed form (ca. 39% yield among clearly resolved motifs, Fig. 3f ). According to the height profile analyses ( Supplementary Fig. S1 ), objects slightly lower (3–4 nm) than SA were observed in the jaws, which is consistent with the expected thickness of IgG. The closing of nanomechanical DNA origami is completely chemoselective, and, therefore, visual discrimination of coexisting proteins in a solution is possible using a mixture of differently shaped and modified origami devices. To demonstrate this concept, we prepared a second DNA origami device, 'DNA origami forceps', which have very similar jaws to DNA pliers but with an extra finger-hole-like structure at the other end of the levers (lower, Fig. 2a ). Biotinylated DNA forceps (white arrows) and FAM-modified DNA pliers (yellow arrows) were separately annealed and mixed together in a 1:1 ratio (left, Fig. 3g ). When SA was added to the mixture (right), biotinylated DNA forceps selectively pinched SA tetramers and adopted the parallel closed form (69% yield), whereas FAM-modified DNA pliers remained intact throughout the process. Detection of metal ions by zipping mechanism Although selective pinching and detection of a target molecule was successful using protein–ligand bindings, among the strongest of all biological interactions, single-molecule pinching of other targets that bind more weakly is usually difficult. A zipping mechanism involving multiple binding events is a second detection mechanism available from the present nanomechanical DNA origami devices and is appropriate for such targets ( Fig. 4 ). Here multiple elements that bind together in the presence of the target are introduced to each of the levers, cooperatively triggering selective closure of the origami devices. Na + ion sensing by DNA origami devices utilizes G-quadruplex formation ( Fig. 4a ), which has been popularly used in spectroscopic detection systems for metal ions [36] . A 12-nucleotide human telomere sequence (5′-TAGGGTTAGGGT-3′; a Telomere Element, TeloE) was attached to the 3′-ends of the staple strands placed at the four sites on each of the levers, spaced every three helical turns on the same side of the fulcrum (sites a , b , c , and d ). This 12-nucleotide sequence is known to dimerize in the presence of Na + by forming an antiparallel G-quadruplex motif and thus acts as a zipper element [37] . The effects of salt on the form of the origami devices were first examined for DNA pliers without any TeloE modification ( Fig. 4b ). On addition of Na + to the solution (final concentration, 200 mM), the population of antiparallel DNA pliers significantly increased from 16% in the solution containing 12.5 mM Mg 2+ alone (top left) to 46% (top right), whereas the percentage of DNA pliers in the cross form decreased ( Fig. 4c ). This change probably occurred because Mg 2+ , which neutralizes phosphates and stabilizes the X-structure of the four-way junction, was partially replaced with the less efficient Na + . The effect of Na + addition on DNA pliers bearing four TeloE (sites a , b , c , and d ) on each lever was quite dramatic. In AFM measurements, almost 64% of the pliers were in parallel closed form, 19% were in antiparallel form, and only 6% were in cross form (bottom left in Fig. 4b ). The yield of parallel closed form clearly correlated to the amount of introduced TeloE and the Na + concentration. The yields of parallel pliers for the motif with one TeloE at site a , with two TeloE at sites a and b , and with three TeloE at sites a , b , and c were 36%, 45%, and 54%, respectively ( Fig. 4c ). For the motif with four TeloE, the yield of parallel pliers correlated almost linearly with Na + concentration up to 100 mM and was approximately saturated thereafter (see Supplementary Fig. S2 ). Buffer exchange of the solution to remove Na + from the system completely opened the parallel closed DNA pliers, as expected (bottom right in Fig. 4b , iv). Fluorescence spectra have shown that Na + -triggered zipping of DNA pliers through G-quadruplex formation proceeds efficiently in solution ( Fig. 4d ) but is rather slow compared with SA-biotin systems. It took 2–3 h to reach equilibrium (20% enhancement of FAM and 52% quenching of TXR emission) after Na + addition, according to the time course of the quenching of TXR emission (inset). Buffer exchange using ultrafiltration resulted in backward transition of the emission to the initial level. The final FAM emission was 80% of the initial intensity, and that of TXR was 89%. The TeloE sequence is known to dimerize in the presence of K + as well, although the dimer is a mixture of two species, parallel and antiparallel G-quadruplex motifs [38] . Selective closure of DNA pliers was also observed with K + addition ( Fig. 4c ). Representing the higher stability of the G-quadruplex containing K + ( T m values for TeloE dimer in the presence of 100 mM K + and Na + are 54 and 42 °C, respectively, data not shown), the yields of parallel pliers were slightly higher than in the systems with corresponding amounts of Na + ( Supplementary Fig. S2 ). In a similar manner to Na + or K + , Ag + ions can be detected by a zipping mechanism by using Ag + -mediated selective stabilization of C–C mismatches ( Fig. 4e ) [39] . Four pairs of complementary DNA elements that involve two C–C mismatches in a 14-mer sequence were attached to each of the levers, as with TeloE. As shown in Figure 4f , almost 47% of DNA pliers were in parallel closed form after the addition of Ag + to the solution. Detection of small molecules by unzipping mechanism Unzipping, which is the reverse process of the zipping mechanism, is the third detection mechanism of the present nanomechanical DNA origami devices ( Fig. 5 ). The zipper elements for this mechanism were designed to bind together at the initial stage and selectively unbind in the presence of target molecules. As shown in Figure 5a , the presence of human micro RNA can be clearly detected using origami devices by employing an unzipping mechanism. For example, 23-mer sequences complementary to miR20 were attached to the four sites for zipper elements in one of the levers of DNA pliers. The other lever was modified with partially complementary 10-mer sequences. DNA pliers bearing these elements were directly annealed into the parallel closed form in the absence of the target. The 13-mer sequences in the 3′ end of the 23-mer elements (red nucleotides in Fig. 5a ) were left single-stranded to serve as a toehold to trigger selective strand displacement by the target. AFM measurements with increasing numbers of preclosing zipper-element pairs from one to four, just after the annealing of DNA pliers, revealed that at least three zipper-element pairs are necessary to obtain sufficient (around 80%) preclosing ( Supplementary Fig. S3 ). Figure 5c shows selective detection of miR20 achieved using a 1:1 mixture of miR20-targeting DNA pliers and miR16-targeting DNA forceps with four preclosing zipper-element pairs. The addition of miR20 to the mixture selectively opened the DNA pliers (shown in blue bars), whereas the DNA forceps persisted in the parallel closed form (red bars). Selective detection of miR16 using the same 1:1 mixture was also possible ( Supplementary Fig. S4 ). Unzipping of dual dye-labelled DNA pliers in solution was successfully monitored by fluorescence measurements, as shown in Figure 5d . Nearly 87% enhancement of TXR emission and 16% quenching of FAM emission were observed within 4 h after the addition of the target under room temperature. A unique advantage of the unzipping mechanism is that different kinds of zipper elements can be introduced into one origami device to work together as an AND logic gate. For example, DNA pliers bearing two miR20-targeting elements (at sites a and c ) and two miR16-targeting elements (at b and d ) did not open until both targets (miR20 AND miR16) were added to the solution ( Fig. 5e ). Origami devices can therefore handle multiple targets within a single device molecule, which may not be easily achievable with simple DNA tweezers. The unzipping mechanism is also appropriate for the detection of small molecules using zipper elements based on DNA (or RNA) aptamers ( Fig. 5b ). When ATP-aptamer-based elements, which bind to two ATP molecules by forming an intrastrand stem-loop structure [40] , [41] , were attached to DNA pliers in combination with corresponding closer elements, 45% of the parallel closed pliers initially formed after annealing were unzipped after the addition of ATP to the solution and were imaged as cross or antiparallel forms ( Fig. 5f ). As expected, the addition of GTP to the solution did not trigger unzipping of the parallel closed pliers. We have successfully applied nanomechanical DNA origami devices to construct visual 'single-molecule beacons' that can detect various targets of a wide range of molecular weights, from metal ions (a few tens of Da) to proteins (hundreds of kDa), at molecular resolution using the same platform. Each of the detection mechanisms we have described—pinching, zipping, or unzipping—for the targets of interest can be freely chosen and used orthogonally on differently shaped origami devices in a single mixture. Comparison between the zipping experiments with Na + and TeloE ( Fig. 4c ) and preclosure of miR20-triggered unzipping systems ( Supplementary Fig. S3 ) may hint at the border between targets appropriate for pinching and those require zipping. When only one zipper-element pair was introduced into DNA pliers, Na + with one TeloE gave ca. 40% closure of DNA pliers. In contrast, the yield of preclosed DNA pliers with only one preclosing zipper-elements pair was as low as 15% (whereas the parallel fraction without any zipper element was around 6%). Increasing the number of zipper-element pairs to two resulted in almost the same yield, around 50%, for both systems. Thus, the border should not be far from these zipper elements. The melting temperature of the TeloE dimer in the presence of 100 mM Na + is 42 °C, whereas the melting temperature for the 10-bp complementary part of the miR20 targeting elements is 31 °C under the conditions employed in the study (12.5 mM Mg 2+ and 4 nM strand concentration, data not shown) or Δ G ° 37 =−11.04 kcal mol −1 (1 M Na + ) [42] . The maximum yield of parallel form in a solution containing a single kind of DNA origami device was ~80%, even for the preclosed DNA pliers used in unzipping systems, which were directly annealed into the closed form whereas the whole lever structure was in the folding process ( Supplementary Fig. S3 ). This maximum yield is rather low compared with the ~90% folding yield reported for simple rectangular DNA origami [18] , but it is still high considering the relatively small number of linkages, including an unfavourable parallel four-way junction, joining the two levers. The observation of origami devices using AFM is a completely single-molecule method. Therefore, the theoretical detection limit of the systems should be exceedingly small, if the reaction volume is further reduced with the aid of microfluidics and MEMS technology. For example, a 4nM solution of DNA origami devices, a typical condition used in the present study, corresponds to 1 origami device molecule in every 0.4 femtolitre (=μm 3 ), which contains 2 target molecules for SA and IgG detection, 50 molecules for 200 nM miRNA, or 2,500 atoms for 10 μM Ag + . Moreover, almost any kind of protein or small molecule can be a target of DNA origami devices by inverting the polarity of the pinching systems from an antigen-modified origami device/antibody combination to an antibody-modified origami device/antigen combination. Taking advantage of the rather large size of the origami devices, the capture and detection of whole virus capsids is feasible too [43] . The development of allosteric metaenzymes by attachment of another functional nanomaterial such as an enzyme to the other end of the levers, enabling the switching of their activity by mechanical movement, would be another interesting application of DNA pliers. Such metaenzymes may provide an extra detection pathway for the structural changes of DNA origami devices: chemical signal amplification, which is popularly employed today, for example, in enzyme immunoassays. The present system may be a first step toward powerful tools in future studies of various nano-biochemical interactions. Materials Staple DNA strands and dye-labelled staples were purchased from Sigma Genosys and used without further purification. Biotin-TEG- and FAM-modified anchor strands were chemically synthesized using the appropriate CPG columns (Glen Research) and were purified by reverse-phase HPLC. AFM imaging was performed on a SPA-300HV system (SII). Preparation of nanomechanical DNA origami devices Detailed structures of nanomechanical DNA origami devices used in the present study are shown in Supplementary Figures S5–S10, and the sequences of the staple strands are shown in Supplementary Tables S1–S3 . The formation of DNA origami devices was accomplished with M13mp18 ssDNA (4 nM, Takara), staples, and anchor strands or zipper elements (16 nM for each strand) in a solution containing Tris (40 mM), acetic acid (20 mM), EDTA (10 mM), and magnesium acetate (12.5 mM, 1×TAE/Mg buffer, 50 μl). This mixture was cooled from 90 to 25 °C at a rate of −1.0 °C min −1 using a PCR thermal cycler to anneal the strands. Induction of the shape transitions After excess staples and anchors were removed from the mixture using an ultrafiltration microtube (Amicon Ultra 0.5 ml–100 K, Millipore), 2 eq. (or 1 eq. for fluorescent measurements) of SA to DNA origami devices (final concentration 4 nM) was added to the solution and immediately subjected to AFM measurement. The selective release of SA via strand displacement was performed using 10 eq. of unset strands at room temperature for 2 h. Pinching of IgG was performed identically to SA pinching, except that the mixture was incubated at room temperature for 24 h before AFM imaging. The closing of DNA pliers using a G-quadruplex zipper was initiated by adding 1/10 volume of 2 M NaCl to the origami solution. The post-opening of DNA pliers by buffer exchange was achieved by concentrating the mixture with the ultrafiltration microtube and re-suspending it in 1×TAE/Mg 2+ buffer three times over 1 h at room temperature (the calculated reduction factor of Na + was 1/11,000). The sensing of K + and Ag + was done in a similar manner, but 1X TA/Mg 2+ buffer was used. The final concentration of KCl was 100 mM, and the concentration of AgNO 3 was 10 μM. The unzipping of preclosed miRNA-targeting DNA pliers was done in the presence of target miRNA (200 nM, 12.5 eq. to each zipper element) at room temperature overnight. The detection of ATP was performed using the appropriate zipper elements and 1 mM ATP. After ATP was added to the solution of DNA pliers, the mixture was cooled from 37 to 25 °C at a rate of −1.0 °C min −1 three times using a PCR thermal cycler. AFM imaging A mixture containing DNA origami devices and the target (3 μl) was deposited on freshly cleaved mica; extra 1×TAE/Mg 2+ buffer (200 μl) was added; and imaging was performed in the fluid DFM scanning mode with a BL-AC40TS tip (Olympus). Typical zoom-out images are shown in Supplementary Figures S11–S18 . DNA origami devices in an image were counted as the cross form, when both of the ends were clearly separated AND the levers around the fulcrum were clearly not laid in parallel. They were counted as the parallel form when at least one of the ends was clearly identified to be in head-to-head (the end of a lever close to the concavity) or tail-to-tail (the opposite end of the lever) contact, or into antiparallel form when head-to-tail contact was clearly observed for at least one of the ends. Devices not in any of the above conditions were counted as unclear motifs. The classification was confirmed by at least three persons. Counted numbers of the motifs for each experiment are shown in Supplementary Tables S4–S14 . Fluorescence measurements A total of 500 μl of doubly dye-labelled DNA origami solution was annealed and concentrated to 50 μl using an ultrafiltration microtube. The final concentration of DNA pliers was 40 nM. The excitation wavelengths for the FAM and TXR spectra were 450 and 550 nm, respectively. How to cite this article: Kuzuya, A. et al . Nanomechanical DNA origami 'single-molecule beacons' directly imaged by atomic force microscopy. Nat. Commun. 2:449 doi: 10.1038/ncomms1452 (2011).